Controllable synthesis of molybdenum tungsten disulfide alloy for vertically composition-controlled multilayer The effective synthesis of two-dimensional transition metal dichalcogenides alloy is essential for successful application in electronic and optical devices based on a tunable band gap. Here we show a synthesis process for Mo 1− x W x S 2 alloy using sulfurization of super-cycle atomic layer deposition Mo 1− x W x O y . Various spectroscopic and microscopic results indicate that the synthesized Mo 1− x W x S 2 alloys have complete mixing of Mo and W atoms and tunable band gap by systematically controlled composition and layer number. Based on this, we synthesize a vertically composition-controlled (VCC) Mo 1− x W x S 2 multilayer using five continuous super-cycles with different cycle ratios for each super-cycle. Angle-resolved X-ray photoemission spectroscopy, Raman and ultraviolet–visible spectrophotometer results reveal that a VCC Mo 1− x W x S 2 multilayer has different vertical composition and broadband light absorption with strong interlayer coupling within a VCC Mo 1− x W x S 2 multilayer. Further, we demonstrate that a VCC Mo 1− x W x S 2 multilayer photodetector generates three to four times greater photocurrent than MoS 2 - and WS 2 -based devices, owing to the broadband light absorption. The band gap modulation of two-dimensional (2D) transition metal dichalcogenides (TMDCs) has been intensively studied, because of their various applications in optoelectronic devices such as photodiodes, phototransistors and solar cells [1] , [2] , [3] . It is well known that the band gap of 2D TMDCs is dependent on the number of layers [4] , [5] , [6] . In addition, alloying 2D TMDCs through the synthesis of Mo 1− x W x S 2 , Mo 1− x W x Se 2 or MoS 2 x Se 2(1− x ) , for example, is another way of practically modulating the band gap. This is an effective approach because of the good thermodynamic stability at room temperature of the alloys, as predicted by theoretical calculations [7] , [8] , [9] , [10] , [11] , [12] , [13] , [14] . Furthermore, recent studies have shown that a vertically composition-controlled (VCC) 2D TMDCs multilayer is feasible for the high performance optoelectronic devices due to functionality of interlayer such as interlayer transition [15] , [16] , [17] , [18] , [19] , [20] , [21] , [22] . However, the reported synthesis processes for 2D TMDCs alloy and VCC 2D TMDCs multilayer, such as exfoliation, chemical vapor deposition and transfer, are limited in respect of systematic control of the composition and the number of layers, and clean interface for strong interlayer coupling [9] , [11] , [21] , [23] . Hence, an improved synthesis process for 2D TMDCs alloy and VCC 2D TMDCs multilayer is highly required. Atomic layer deposition (ALD), which is based on surface reactions between precursors and reactants, has benefits such as high purity, thickness control on the atomic scale and large area uniformity [24] , [25] . In particular, it is suitable for the synthesis of alloy thin films with precisely controlled composition using the super-cycle method [26] , [27] , [28] . In addition, a continuous super-cycle process with different cycle ratios can produce a VCC multilayer with a clean interface [29] . In a previous report, we have shown that atomically thin, layer-controlled and wafer-level uniform 2D WS 2 can be synthesized by sulfurization of ALD WO 3 thin films [30] . Here we report a synthesis method of Mo 1− x W x S 2 alloys by sulfurization of super-cycle ALD Mo 1− x W x O y alloy thin films. Using this method, we systematically control the composition and layer number (from mono- to tri-layers) of Mo 1− x W x S 2 alloys by controlling the cycle ratio between the ALD MoO x and WO 3 . The bandgaps of the Mo 1− x W x S 2 alloys are precisely controlled as functions of the composition and layer numbers of each respective alloy, as measured based on the photoluminescence (PL) spectra. Scanning transmission electron microscopy (STEM) shows the mixing of Mo and W atoms with shared metal atom sites in monolayer Mo 1− x W x S 2 alloy. Furthermore, we develop a process to synthesize a VCC Mo 1− x W x S 2 multilayer using a sequential super-cycle ALD process—specifically, 5 continuous super-cycles of ALD with different cycle ratios for each super-cycle. Ultraviolet–visible spectrophotometer analysis shows that the synthesized VCC Mo 1− x W x S 2 multilayer has stronger interlayer coupling than that of a stacked VCC Mo 1− x W x S 2 multilayer fabricated by the individual transfer of each monolayer Mo 1− x W x S 2 alloy. This can be attributed to the clean interface between each layer in the synthesized sample [15] , [21] . MoS 2 synthesis Previously, we reported the synthesis of WS 2 using sulfurization of ALD WO 3 thin film with a one-step sulfurization process at 1,000 °C (ref. 30 ). These synthesized WS 2 exhibit smooth and continuous surfaces with layer controllability from mono- to tetra-layer. Based on this result, we sulfurized ALD MoO x thin film (nine cycles, optimization of ALD MoO x is represented in Supplementary Fig. 1 ) using a one-step sulfurization process at 1,000 °C (see experimental section) to synthesize MoS 2 . 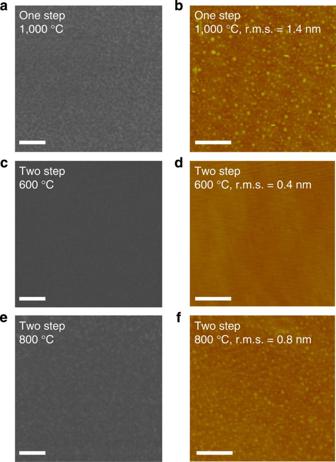Figure 1: Sulfurization of MoOxthin films. (a) SEM and (b) AFM images of sulfurized MoOxthin film using one-step sulfurization process at 1,000 °C. SEM and AFM images of sulfurized MoOxthin film using two-step sulfurization process with first-sulfurization temperatures of (c,d) 600 and (e,f) 800 °C, respectively. Scale bars, (a,c,e) 200 nm and (b,d,f) 0.5 μm. Figure 1a,b comprises scanning electron microscope (SEM) and atomic force microscopy (AFM) images of sulfurized MoO x thin film using the one-step sulfurization process at 1,000 °C. In contrast to WS 2 , however, the MoS 2 shows a rough and non-continuous surface, and the measured root mean square (r.m.s.) is much larger (1.4 nm) than that of the SiO 2 substrate (0.37 nm). We surmise that this discrepancy between the MoO x and WO 3 thin films sulfurized at the same temperature (1,000 °C) is caused by the relatively lower vaporization temperature of MoO x ( ∼ 700 °C) in comparison with WO 3 (over 1,100 °C) [31] . In other words, the MoO x is vaporized before the conversion to MoS 2 is complete, resulting in a rough surface. Figure 1: Sulfurization of MoO x thin films. ( a ) SEM and ( b ) AFM images of sulfurized MoO x thin film using one-step sulfurization process at 1,000 °C. SEM and AFM images of sulfurized MoO x thin film using two-step sulfurization process with first-sulfurization temperatures of ( c , d ) 600 and ( e , f ) 800 °C, respectively. Scale bars, ( a , c , e ) 200 nm and ( b , d , f ) 0.5 μm. Full size image Therefore, we examined the effect of sulfurization temperature on the roughness of the sulfurized ALD MoO x thin film. To achieve this, we conducted a two-step sulfurization process, which consists of a low-temperature first step for the sulfurization of the MoO x and a high-temperature second step to enhance the MoS 2 crystallinity. The first-sulfurization temperatures were set to lower (600 °C) and higher (800 °C) temperatures than the vaporization temperature of MoO x (700 °C), while the second-sulfurization temperature and process time were kept at 1,000 °C and 150 min, respectively (see Methods section). The roughness of the sulfurized MoO x thin films in accordance with first-sulfurization temperature was then compared using SEM and AFM ( Fig. 1c–f ). Figure 1c,e shows SEM images of the sulfurized MoO x thin films for first-sulfurization temperatures of 600 °C and 800 °C, respectively. The sulfurized MoO x thin film at a first-sulfurization temperature of 600 °C has a smooth and continuous surface, while the MoO x thin film sulfurized at a first-sulfurization temperature of 800 °C has a rough and non-continuous surface. AFM analyses ( Fig. 1d,f ) illustrate the variations in the roughness of the sulfurized MoO x thin films more clearly, which is due to the differing first-sulfurization temperatures. The r.m.s. value for the MoS 2 sulfurized at 600 °C is very low ( ∼ 0.4 nm) and is close to the r.m.s. value of the SiO 2 substrate (0.37 nm). In contrast, the r.m.s. value of the MoS 2 in the 800 °C case is relatively high (0.8 nm). As a result, a first-sulfurization temperature of 600 °C results in MoS 2 with uniform and continuous surfaces, due to the fact that the first-sulfurization temperature is lower than the vaporization temperature of MoO x , as we assumed. Based on this result, we used a two-step sulfurization process with a 600 °C first-sulfurization temperature to synthesize continuous MoS 2 and Mo 1− x W x S 2 alloys. Next, layer-number-controlled MoS 2 was synthesized utilizing the two-step sulfurization process described above. 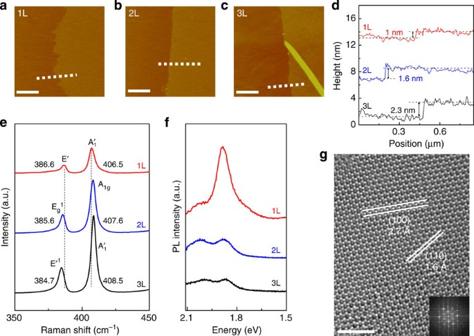Figure 2: Characterization of MoS2. (a–c) AFM images and (d) height profiles (along with white dashed line in AFM images) of transferred MoS2on SiO2substrate for 1l, 2l and 3l thickness, respectively. Scale bars, 0.5 μm. (e) Raman spectra and (f) PL spectra for 1l (red), 2l (blue) and 3l (black) MoS2on SiO2substrate. (g) HRTEM image of 1l MoS2at a selected region and (inset) FFT pattern. Scale bars, 2 nm. Figure 2a–d shows the AFM images and height profiles of the transferred MoS 2 , which were synthesized by sulfurizing MoO x thin films deposited by 6, 9 and 12 ALD cycles. The measured thicknesses of the synthesized MoS 2 were ∼ 1, 1.6 and 2.3 nm for 6, 9 and 12 MoO x ALD cycles, respectively. These thicknesses correspond to mono-, bi- and tri-layer (1, 2 and 3l) MoS 2 , considering that the height of 1l MoS 2 on SiO 2 is ∼ 1 nm and the spacing between the first and second MoS 2 layers is ∼ 0.6 nm (refs 3 , 4 ). As reported previously, the larger AFM-measured spacing between the first MoS 2 layer and the substrate, compared with that between the MoS 2 layers, is caused by the effect of distinct tip–sample and tip–substrate interactions [3] , [30] , [32] . Also, the apparent colour gains of the transferred 1, 2 and 3l MoS 2 are observed in optical microscopy (OM) images ( Supplementary Fig. 2 ). It should be noted that the MoS 2 is not formed in the case of an ALD MoO x thin film with an ALD cycle number of <3 ( Supplementary Fig. 3 ). This is attributed to a nucleation delay during the initial growth of the MoO x , and similar behaviour was observed during the synthesis of WS 2 by sulfurization of ALD WO 3 (ref. 30 ). After the nucleation delay, 1l of MoS 2 is formed by the sulfurization of each three-cycle ALD MoO x thin film sample ( ∼ 0.8−0.9 nm in thickness). This observation agrees with a previous report, where ∼ 1 nm of MoO x film transformed into a 1l MoS 2 via sulfurization [33] . The stoichiometry calculated from X-ray photoemission spectroscopy (XPS) result is 2 (S/Mo) as shown in Supplementary Fig. 4 . As a result, we can systematically control the layer number of MoS 2 by controlling the ALD MoO x cycle number. Figure 2: Characterization of MoS 2 . ( a – c ) AFM images and ( d ) height profiles (along with white dashed line in AFM images) of transferred MoS 2 on SiO 2 substrate for 1l, 2l and 3l thickness, respectively. Scale bars, 0.5 μm. ( e ) Raman spectra and ( f ) PL spectra for 1l (red), 2l (blue) and 3l (black) MoS 2 on SiO 2 substrate. ( g ) HRTEM image of 1l MoS 2 at a selected region and (inset) FFT pattern. Scale bars, 2 nm. Full size image The MoS 2 were further characterized using Raman, PL and high-resolution TEM (HRTEM). The Raman spectra ( λ exc =532 nm) for 1, 2l and 3l MoS 2 are shown in Fig. 2e . The MoS 2 exhibit in-plane and out-of-plane vibrations modes at 386.6 and 406.5 cm −1 (E′ and A′ 1 ) for the 1l, 385.6 and 407.6 cm −1 (E g 1 and A 1g ) for 2l, and 384.7 and 408.5 cm −1 (E′ 1 and A′ 1 ) for 3l (ref. 34 ). From the Raman spectra, we calculated the relative peak distance between the in-plane and out-of-plane modes, which is closely related to the layer number of the MoS 2 due to the softening in the in-plane and stiffening in the out-of-plane mode frequencies, with increasing layer numbers [35] , [36] . The calculated relative peak distances are 19.9, 22 and 23.8 cm −1 for the 1, 2 and 3l samples, respectively, which are in good agreement with previously reported values for synthesized MoS 2 (refs 37 , 38 , 39 ). The PL spectra dependence on the layer number of the MoS 2 is shown in Fig. 2f . The spectrum of the 1l MoS 2 shows PL peaks at 1.89 eV and 2.01 eV, which are correlated to the A 1 and B 1 direct excitonic transitions of the MoS 2 , respectively. With increasing layer number, weak PL peaks are observed at 1.87 eV and 2.00 eV for the 2l, and 1.86 eV and 1.99 eV for the 3l. The red shift and low intensity of the PL peaks with increasing layer number is due to the band gap transition from direct to indirect, which is consistent with the dependency of the PL peak on the layer number [4] , [5] , [6] , [40] . These Raman and PL results again confirm the layer controllability of MoS 2 using the ALD process. Figure 2g is an HRTEM image for the synthesized 1l MoS 2 . The MoS 2 shows a honeycomb-like structure with lattice spacing of 0.27 nm and 0.16 nm for the (100) and (110) planes, respectively. In addition, sixfold coordination symmetry is observed in the fast Fourier transformation (FFT) image (inset of Fig. 2g ). The approximate domain size is 10−20 nm, similar to that of previously reported synthesized MoS 2 and WS 2 using the sulfurization of MoO x and WO 3 thin films [30] , [41] . Mo 1− x W x S 2 alloy synthesis A super-cycle ALD-based Mo 1− x W x S 2 alloy synthesis process was developed based on the synthesis processes for 2D MoS 2 (this study) and WS 2 (previous study) [30] . The overall synthesis scheme for the Mo 1− x W x S 2 alloy is illustrated in Fig. 3a . First, we conducted 10 cycles of WO 3 ALD to address the nucleation delay of the ALD WO 3 (ref. 30 ) (not shown in Fig. 3a ). Subsequently, one super-cycle ALD process consisting of n cycles of ALD MoO x and m cycles of ALD WO 3 was conducted and the deposited Mo 1− x W x O y alloy thin films were sulfurized. We used varying cycles for MoO x ( n ) and WO 3 ( m ) in one super-cycle to deposit 0.8−0.9-nm-thick composition-controlled Mo 1− x W x O y alloy thin films to create a 1l Mo 1− x W x S 2 alloy. This was based on the growth rate of ALD MoO x (2.7 Å per cycle) and WO 3 (0.9 Å per cycle), as shown in Supplementary Table 1 . 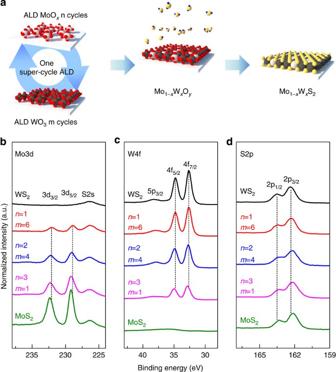Figure 3: Synthesis and XPS of Mo1−xWxS2alloy. (a) Synthesis procedure of super-cycle ALD for Mo1−xWxS2alloy. XPS measurements for (b) Mo3d, (c) W4f and (d) S2p core levels in the 1l Mo1−xWxS2alloy with differentnandmnumbers in one super-cycle. All measured XPS results are normalized by S2p3/2peak intensity. Figure 3b–d shows the XPS spectra of the 1l MoS 2 , 1l WS 2 and sulfurized Mo 1− x W x O y alloy thin films with different n and m numbers in one super-cycle. All measured XPS results were normalized by S2p 3/2 peak intensity and calibrated to the C1s peak at 285 eV. With increasing n / m ratio, the intensity of the Mo3d peaks increased, while the W5p 3/2 and W4f peaks decreased. Furthermore, the peak positions for Mo3d and W4f gradually shifted to higher binding energies, from 232.2 eV and 229.1 eV to 232.5 eV and 229.4 eV for Mo3d 3/2 and Mo3d 5/2 , respectively, and from 34.8 eV and 32.6 eV to 35.0 eV and 32.8 eV for W4f 5/2 and W4f 7/2 , respectively. In addition, the S2p peaks shifted to lower binding energies, from 163.5 eV and 162.4 eV to 163.3 eV and 162.2 eV for S2p 1/2 and S2p 3/2 , respectively. This small shift in peak position is attributed to the enhanced electron attraction strength of S and the reduced electron attraction strength of W, following increased Mo content due to smaller electronegativity of Mo (2.16) than that of W (2.36) as previously reported [7] . It is noteworthy that the Mo 6+ 3d 3/2 peak, which is attributed to the Mo–O bonding, is not observed in the Mo3d spectra; this indicates the absence of O species. Figure 3: Synthesis and XPS of Mo 1− x W x S 2 alloy. ( a ) Synthesis procedure of super-cycle ALD for Mo 1− x W x S 2 alloy. XPS measurements for ( b ) Mo3d, ( c ) W4f and ( d ) S2p core levels in the 1l Mo 1− x W x S 2 alloy with different n and m numbers in one super-cycle. All measured XPS results are normalized by S2p 3/2 peak intensity. Full size image We calculated the Mo, W and S concentrations from the XPS results for the Mo3d, W4f and S2p peaks, respectively, to examine the Mo 1− x W x S 2 alloy composition. Table 1 presents the calculated concentration and W composition, x . The calculated x value is dependent on the n and m numbers in a single super-cycle, and yields x =0.8 for n =1 and m =6, x =0.6 for n =2 and m =4, and x =0.3 for n =3 and m =1. Also, the calculated stoichiometry is 2 (S/(Mo+W)). This shows that the W composition ( x ) in the Mo 1− x W x S 2 alloys can be systematically modulated by changing the values of n and m in one super-cycle. Table 1 Calculated composition of Mo 1− x W x S 2 . Full size table The synthesized composition-controlled Mo 1− x W x S 2 alloy from super-cycle ALD Mo 1− x W x O y alloy thin films were characterized using AFM, Raman and PL, as shown in Fig. 4 . The AFM images and height profiles of the transferred Mo 1− x W x S 2 alloys are represented in Fig. 4a−d and they show good uniformity and continuity (also see OM images in Supplementary Fig. 5 ). The measured thicknesses of the Mo 0.2 W 0.8 S 2 , Mo 0.4 W 0.6 S 2 and Mo 0.7 W 0.3 S 2 alloys were all ∼ 1 nm, corresponding to the 1l thickness of Mo 1− x W x S 2 alloy. Furthermore, 2 and 3l Mo 1− x W x S 2 alloys can be synthesized using two- and three-super-cycle ALD Mo 1− x W x O y alloy thin films ( Supplementary Fig. 6 ). As a result, our super-cycle ALD-based Mo 1− x W x S 2 alloy synthesis process can systematically control the layer number, as well as the composition of the resultant alloys through manipulation of the super-cycle ALD process. 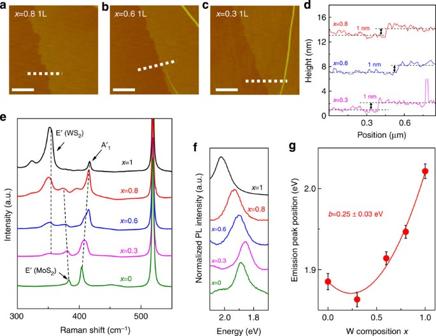Figure 4: Characterization of Mo1−xWxS2alloy. (a–c) AFM images and (d) height profiles (along with white dashed line in AFM images) of transferred 1l Mo1−xWxS2alloy on SiO2substrate forx=0.8, 0.6 and 0.3, respectively. Scale bars, 0.5 μm. (e) Raman spectra and (f) PL spectra for 1l Mo1−xWxS2alloy on SiO2substrate forx=1, 0.8, 0.6, 0.3 and 0. (g) PL peak position versus W composition (x) graph. Error bars represent s.d. of PL peak position in five-times repeatedly synthesized Mo1−xWxS2alloy. Figure 4: Characterization of Mo 1− x W x S 2 alloy. ( a – c ) AFM images and ( d ) height profiles (along with white dashed line in AFM images) of transferred 1l Mo 1− x W x S 2 alloy on SiO 2 substrate for x =0.8, 0.6 and 0.3, respectively. Scale bars, 0.5 μm. ( e ) Raman spectra and ( f ) PL spectra for 1l Mo 1− x W x S 2 alloy on SiO 2 substrate for x =1, 0.8, 0.6, 0.3 and 0. ( g ) PL peak position versus W composition ( x ) graph. Error bars represent s.d. of PL peak position in five-times repeatedly synthesized Mo 1− x W x S 2 alloy. Full size image Figure 4e shows the Raman spectra of composition-controlled 1l Mo 1− x W x S 2 alloys. The 1l WS 2 ( x =1) exhibits first-order modes: out-of-plane (A′ 1 ) and in-plane (E′) modes at 417 cm −1 and 357 cm −1 , respectively, and a second-order mode: 2LA(M) at 353 cm −1 (ref. 30 ). The A′ 1 mode shifts to a lower frequency with decreasing W composition, while the E′ mode related to WS 2 does not noticeably shift with the reduction of intensity. In addition, an E′ mode related to MoS 2 appear at x =0.8 and shifted to a higher frequency with a reduction in W composition. The specific peak position dependency on W composition is represented in Supplementary Fig. 7 , and the W composition dependence of the Raman spectra of the 1l Mo 1− x W x S 2 alloy is consistent with previous reports [7] , [8] , [9] . The normalized PL spectra of the composition-controlled 1l Mo 1− x W x S 2 alloys are shown in Fig. 4f , also the x values versus the average PL peak positions and s.d. of five-times repeatedly synthesized 1l Mo 1− x W x S 2 alloys are plotted in Fig. 4g . As the value of x increased from 0 to 1, the averaged PL peak position initially decreases from 1.885 to 1.863 eV, and then gradually increases to 2.021 eV. This non-linear PL peak position behaviour with changing x is the so-called ‘bowing effect’, and has also been reported for other semiconducting alloys and exfoliated 1l Mo 1− x W x S 2 alloys [9] , [42] , [43] . The bowing effect in 1l Mo 1− x W x S 2 alloy can be described by the Equation (1), where b is a bowing parameter. After fitting the experimental results as shown in Fig. 4g (red solid curve), a b value of 0.25±0.03 eV was extracted. The extracted b value is comparable to that of the previous experiment (0.25±0.04 eV) and simulation (0.28±0.04 eV) results [9] . Furthermore, the s.d. of the five-times repeatedly synthesized 1l Mo 1− x W x S 2 alloys are small within the range of 0.008 to 0.01, which indicates that the process has good reliability in terms of composition control. Thus, the PL result confirms that we modulate the band gap of the Mo 1− x W x S 2 alloy by reliably controlling the composition. Moreover, the band gap can also be modulated by controlling the layer number (see Supplementary Fig. 8 ). 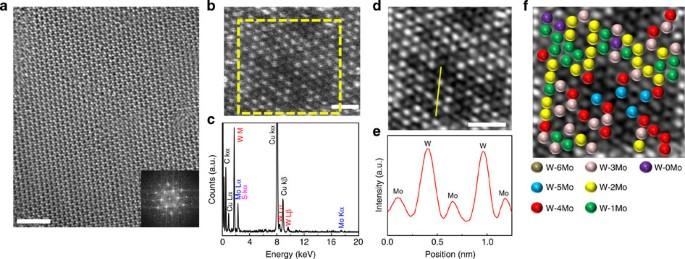Figure 5: Atomic arrangement and mixture of Mo0.4W0.6S2alloy. (a) HRTEM image of 1l Mo0.4W0.6S2alloy at a selected region, and (inset) FFT pattern. Scale bars, 2 nm. (b) STEM-ADF image of 1l Mo0.4W0.6S2alloy at a selected region and (c) corresponding EDX spectrum. Scale bars, 1 nm. (d) Inverse FFT image with masking applied to yellow dashed square region inb. Scale bars, 1 nm. (e) Intensity profile of yellow solid line ind. (f) Coloured W atoms with light brown, blue, red, dark red, yellow, green and violet for six, five, four, three, two, one and zero number of neighbouring Mo atoms. Figure 5a is the HRTEM image of the 1l Mo 0.4 W 0.6 S 2 alloy ( x =0.6). The Mo 0.4 W 0.6 S 2 alloy shows a periodic atomic arrangement with a honeycomb-like structure and sixfold coordination symmetry, similar to the 1l MoS 2 shown in Fig. 2f . To distinguish between the W and Mo atoms in the 1l Mo 0.4 W 0.6 S 2 alloy, we analysed the Mo 0.4 W 0.6 S 2 alloy using STEM annular dark-field and energy dispersive X-ray spectrometry (EDX). Figure 5b is the STEM-ADF image of the 1l Mo 0.4 W 0.6 S 2 alloy. Brighter and less bright spots, which correspond to W and Mo atoms, respectively, are clearly resolved in the ADF image, as previously reported [44] . The calculated Mo/W ratio from the atom count in Fig. 5b is 0.42:0.58, which differs by <5% from the XPS-measured stoichiometry. In addition, the EDX result in Fig. 5c supports the presence of W, Mo and S species in the 1l Mo 0.4 W 0.6 S 2 alloy. To extract a clear intensity difference between the W and Mo atoms, we performed an inverse FFT by applying a mask to the yellow dashed square region in Fig. 5b . Figure 5d–e shows the inversed FFT image ( Fig. 5d ) and intensity profile ( Fig. 5e ) along with the yellow solid line in Fig. 5d . Although S atoms are not distinguishable in our result as a result of the displacement of S atoms at 200 kV operation voltage by the knock-on mechanism [45] , the W and Mo atoms are clearly observable, confirming that these elements share the metal atom sites [44] . The preference for Mo or W atoms at the neighbouring sites of W atoms is evaluated by degree of alloying that can be calculated by Equation (2) [23] , [44] , Figure 5: Atomic arrangement and mixture of Mo 0.4 W 0.6 S 2 alloy. ( a ) HRTEM image of 1l Mo 0.4 W 0.6 S 2 alloy at a selected region, and (inset) FFT pattern. Scale bars, 2 nm. ( b ) STEM-ADF image of 1l Mo 0.4 W 0.6 S 2 alloy at a selected region and ( c ) corresponding EDX spectrum. Scale bars, 1 nm. ( d ) Inverse FFT image with masking applied to yellow dashed square region in b . Scale bars, 1 nm. ( e ) Intensity profile of yellow solid line in d . ( f ) Coloured W atoms with light brown, blue, red, dark red, yellow, green and violet for six, five, four, three, two, one and zero number of neighbouring Mo atoms. Full size image where P observed is the averaged ratio of number of neighbouring Mo atoms to total neighbouring sites of W atoms, and P random is the total ratio of Mo atoms in the examined layer. Figure 5f represented differently coloured W atoms depending on number of neighbouring Mo atoms: light brown, blue, red, dark red, yellow, green and violet for six, five, four, three, two, one and zero number of neighbouring Mo atoms. The calculated degree of alloying is 99%, which indicate that there is no preference for Mo or W atoms at the neighbouring sites of W atoms and a random mixture of our 1l Mo 1− x W x S 2 alloy. A VCC Mo 1− x W x S 2 synthesis The composition controllability of our ALD-based Mo 1− x W x S 2 alloy synthesis process enables synthesis of a VCC Mo 1− x W x S 2 multilayer with a clean interface, strong interlayer coupling and broadband light absorption. We sulfurized a VCC Mo 1− x W x O y thin film that was deposited by a sequential super-cycle ALD process, so as to synthesize a VCC Mo 1− x W x S 2 multilayer, as shown in Fig. 6a . First, we conducted 20 cycles of WO 3 ALD on a SiO 2 substrate, corresponding to 1l WS 2 . We immediately performed three super-cycles of Mo 1− x W x O y ALD with different super-cycle n and m numbers, in the following order: n =1 and m =6, n =2 and m =4, and n =3 and m =1. Last, we conducted three cycles of MoO x ALD ( n =3) corresponding to 1l MoS 2 . The deposited VCC Mo 1− x W x O y thin film was sulfurized to convert it into a VCC Mo 1− x W x S 2 multilayer. 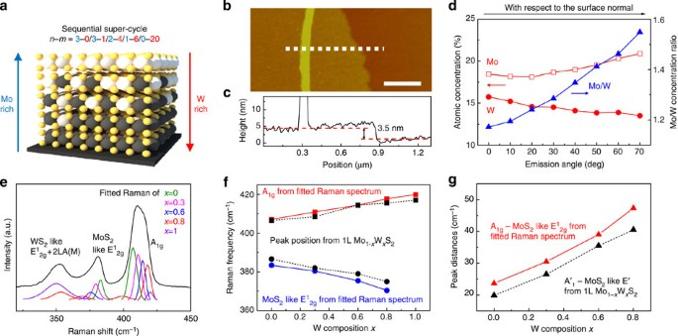Figure 6: Characterization of VCC Mo1−xWxS2multilayer. (a) Sequential super-cycle ALD procedure and schematic structure of a VCC Mo1−xWxS2multilayer. (b) AFM image and (c) height profiles (along with white dashed line in AFM image) for a VCC Mo1−xWxS2multilayer. Scale bars, 0.5 μm. (d) Calculated atomic concentration and relative concentration ratio of Mo and W from ARXPS measurement. (e) Raman spectra for a VCC Mo1−xWxS2multilayer. (f) Raman peak position of A1gand MoS2-like E12gmodes from fitted Raman spectra (red and blue solid line) and from measured Raman spectra of 1l Mo1−xWxS2alloy (black dashed line). (g) Calculated Raman peak distances between A1gand MoS2-like E12gmodes from fitted Raman spectra (red solid line) and from measured Raman spectra of 1l Mo1−xWxS2alloy (black dashed line). Figure 6b,c shows an AFM image and height profile of the transferred VCC Mo 1− x W x S 2 multilayer, with a measured thickness of ∼ 3.5 nm. This thickness, synthesized by five sequential ALD super-cycles, corresponds to a 5l Mo 1− x W x S 2 alloy, which is consistent with each super-cycle result for the 1l Mo 1− x W x S 2 alloy. Figure 6: Characterization of VCC Mo 1− x W x S 2 multilayer. ( a ) Sequential super-cycle ALD procedure and schematic structure of a VCC Mo 1− x W x S 2 multilayer. ( b ) AFM image and ( c ) height profiles (along with white dashed line in AFM image) for a VCC Mo 1− x W x S 2 multilayer. Scale bars, 0.5 μm. ( d ) Calculated atomic concentration and relative concentration ratio of Mo and W from ARXPS measurement. ( e ) Raman spectra for a VCC Mo 1− x W x S 2 multilayer. ( f ) Raman peak position of A 1g and MoS 2 -like E 1 2g modes from fitted Raman spectra (red and blue solid line) and from measured Raman spectra of 1l Mo 1− x W x S 2 alloy (black dashed line). ( g ) Calculated Raman peak distances between A 1g and MoS 2 -like E 1 2g modes from fitted Raman spectra (red solid line) and from measured Raman spectra of 1l Mo 1− x W x S 2 alloy (black dashed line). Full size image The different composition concentrations of the bottom and top layers in the VCC Mo 1− x W x S 2 multilayer were analysed using angle-resolved XPS (ARXPS). Figure 6d shows the calculated atomic and relative concentration ratios of the Mo and W from the ARXPS measurement (ARXPS spectra are shown in Supplementary Fig. 9 ). The Mo concentration increased from 18.6 to 20.9%, while the W concentration decreased from 15.7 to 13.5%, with increasing emission angle from 0 to 70° (red line). The Mo/W concentration ratio increased from 1.17 to 1.55 with increasing emission angle (blue line). Although the exact atomic concentration according to position in the VCC Mo 1− x W x S 2 multilayer cannot be calculated because of the larger depth resolution of the XPS measurement in comparison with the VCC Mo 1− x W x S 2 multilayer thickness, the emission angle dependency of the Mo and W concentration indicates Mo-rich and W-rich concentration in the upper and lower layers of the VCC Mo 1− x W x S 2 multilayer, respectively. As a result, ARXPS shows that the VCC Mo 1− x W x S 2 multilayer has VCC characteristics. Notably, the calculated stoichiometry ratio was 2 (S/(Mo+W)) in all ARXPS results. The formation of Mo 1− x W x S 2 alloy with different compositions in a VCC Mo 1− x W x S 2 multilayer was analysed using Raman spectroscopy. Figure 6e shows the Raman spectrum of a VCC Mo 1− x W x S 2 multilayer, which exhibits strong peaks for A 1g , MoS 2 -like E 1 2g and WS 2 -like E 1 2g +2LA(M) modes. Each Raman peak can be fitted using a Lorentzian function to the Raman spectrum of the Mo 1− x W x S 2 alloy with x =0, 0.3, 0.6, 0.8 and 1. The fitted Raman spectrum was compared with the measured Raman spectrum for the 1l Mo 1− x W x S 2 alloy, with respect to variations in the peak position and peak distances of the A 1g and MoS 2 -like E 1 2g modes, depending on W concentration. The A 1g and MoS 2 -like E 1 2g peak positions from the fitted Raman spectrum are represented in Fig. 6f with the measured Raman peak positions for the 1l Mo 1− x W x S 2 alloy (black dashed line, the same as Supplementary Fig. 7 ). The variation in the fitted Raman peak position with increasing W concentration in the Mo 1− x W x S 2 alloy is the same as the variation in the measured Raman peak position for the 1l Mo 1− x W x S 2 alloy: A 1g shifts to a higher frequency with an increase in W concentration, while the MoS 2 -like E 1 2g modes downshift. Figure 6g shows peak distances between the A 1g and MoS 2 -like E 1 2g modes from the fitted Raman spectrum (red solid line) and measured Raman spectrum of the 1l Mo 1− x W x S 2 alloy (black dashed line), which are 3−4 cm −1 larger than that of the Raman spectrum of the 1l Mo 1− x W x S 2 alloy. This is due to the softening in the MoS 2 -like E 1 2g mode frequency and stiffening in the A 1g mode frequency. Similar behaviour, that is, increasing peak distances with increasing layer number, is also observed in MoS 2 (refs 35 , 36 ) and WS 2 (ref. 30 ) because of the reduced long-range Coulomb interaction between the effective charges, which is induced by an increase in the dielectric screening. These results for the fitted Raman spectra are in good agreement with the dependency of the peak positions on the W composition given by the measured Raman results, and the dependency of the peak distances on layer number in 2D TMDCs. Thus, we can conclude that the fitted Raman spectra show the formation of a Mo 1− x W x S 2 alloy with different compositions in a VCC Mo 1− x W x S 2 multilayer. As a result, it can be stated that the ARXPS and Raman results show the VCC characteristics of a VCC Mo 1− x W x S 2 multilayer. Also, these findings indicate that the vertical interdiffusion of the Mo and W atoms during the sulfurization process have no critically effect on the VCC characteristics. A similar result was observed in a previous report, in that MoO x /WO 3 thin film was converted to MoS 2 /WS 2 without the formation of a Mo 1− x W x S 2 alloy, indicating the limited interdiffusion of Mo and W atoms [46] . Further, it is noteworthy that we verified the validity of ARXPS and Raman measurements as a means of characterizing the VCC Mo 1− x W x S 2 multilayer via characterization of a VCC Mo 1− x W x S 2 multilayer synthesized with a reversed vertical composition profile (see Supplementary Fig. 10 ). Since the interlayer coupling affects interlayer transition [15] , [21] , [47] , [48] , strong interlayer coupling in a synthesized VCC Mo 1− x W x S 2 multilayer was evaluated using comparison of interlayer transition in three difference sample types as shown in Fig. 7a . Sample 1 is a stacked VCC Mo 1− x W x S 2 multilayer fabricated by the transfer of each differently composed Mo 1− x W x S 2 alloy onto glass substrate, while sample 2 is the same as sample 1 but annealed at 200 °C for 15 min in an Ar ambient atmosphere to enhance the interlayer coupling by the removal of residual molecules [21] , [48] . Sample 3 is a transferred VCC Mo 1− x W x S 2 multilayer on glass substrate, which was annealed at 200 °C for 15 min in an Ar ambient atmosphere. Ultraviolet–visible spectrophotometer measurements for samples 1, 2 and 3 ( Fig. 7b ) illustrate that these have broadband light absorption properties due to the sum of the light absorption from the differently composed Mo 1− x W x S 2 alloys. In previous reports, the absorption spectrum of the interlayer transition could be obtained by comparing the intensity difference between the absorption spectra of the weakly interlayer-coupled sample and that of the strongly interlayer-coupled sample [15] , [48] . Based on these reports, we extracted the interlayer transition absorption spectrum by subtracting the absorption spectrum of sample 1 from that of sample 2 and of sample 3, since sample 1 has the weakest interlayer coupling of the three samples as a result of the contamination at the interface caused by the layer transfer process [15] , [21] , [48] . The extracted absorption spectra of the interlayer transition are shown in Fig. 7c . The sample 2–sample 1 spectrum (black solid line) shows a small absorbance peak at 1.87 eV, while the sample 3–sample 1 spectrum (red solid line) shows an absorbance peak that is over five times stronger than the sample 2–sample 1 absorbance peak at the same position. Specific observations on the origin of the absorbance peak position from the interlayer transition (1.87 eV) are described in the Supplementary Information ( Supplementary Fig. 11 ). The stronger absorbance peak of sample 3–sample 1 in comparison with that of sample 2–sample 1 indicates that sample 3 has stronger interlayer coupling compared with sample 2. In other words, a VCC Mo 1− x W x S 2 multilayer based on sequential super-cycle ALD has the strongest interlayer coupling among the three types of samples. We surmise that this strong interlayer coupling results from the absence of a transfer process, which eliminates the incorporation of residual molecules such as H 2 O and organic contaminants [15] , [21] , [47] , [48] . 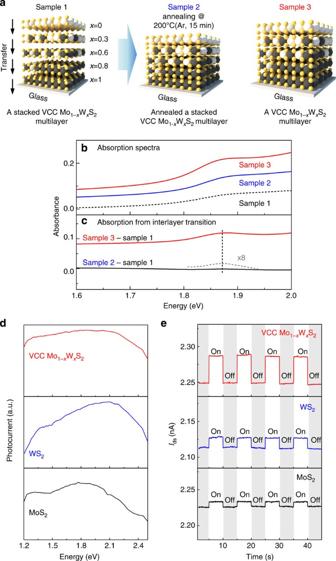Figure 7: Absorbance and photoinduced current of VCC Mo1−xWxS2multilayer. (a) Schematics of three sample types for ultraviolet–visible spectrophotometer measurement. (b) Absorption spectra of sample 1 (black solid line), sample 2 (blue solid line), and sample 3 (red solid line) and (c) extracted absorption spectra of interlayer transition using subtraction of sample 1 from sample 2 (black solid line) and from sample 3 (red solid line). (d) Spectral and (e) time-resolved photocurrent of a VCC Mo1−xWxS2multilayer, 5l WS2and 5l MoS2photodetectors. Figure 7: Absorbance and photoinduced current of VCC Mo 1− x W x S 2 multilayer. ( a ) Schematics of three sample types for ultraviolet–visible spectrophotometer measurement. ( b ) Absorption spectra of sample 1 (black solid line), sample 2 (blue solid line), and sample 3 (red solid line) and ( c ) extracted absorption spectra of interlayer transition using subtraction of sample 1 from sample 2 (black solid line) and from sample 3 (red solid line). ( d ) Spectral and ( e ) time-resolved photocurrent of a VCC Mo 1− x W x S 2 multilayer, 5l WS 2 and 5l MoS 2 photodetectors. Full size image A VCC Mo 1− x W x S 2 multilayer exhibits a broadband light absorption property, as well as strong interlayer coupling. Thus, the VCC Mo 1− x W x S 2 multilayer has promising potential use as an active layer in an efficient photodetector. To evaluate the photoinduced response of the VCC Mo 1− x W x S 2 multilayer, we observed the spectral and time-resolved photocurrent of a VCC Mo 1− x W x S 2 multilayer photodetector and compared it with 5l WS 2 and 5l MoS 2 photodetectors (see the Methods section for details of device fabrication, and see Supplementary Fig. 12 for AFM images of the 5l MoS 2 and WS 2 and their I – V characteristics). Figure 7d shows the dependence of the photocurrent on the illumination energy for the VCC Mo 1− x W x S 2 multilayer, 5l WS 2 , and 5l MoS 2 photodetectors for a voltage drain to source ( V ds ) of 5 V. The continuum power spectral density is represented in Supplementary Fig. 13 . The VCC Mo 1− x W x S 2 multilayer photodetector generates a broadband photoinduced current from 1.2 to 2.5 eV, because of its broadband light absorption property. In contrast, the 5l WS 2 and 5l MoS 2 photodetectors generate narrower photocurrents than the VCC Mo 1− x W x S 2 multilayer, at 1.3 and 2.1 eV for the 5l WS 2 photodetector and 1.2 and 1.8 eV for the MoS 2 device; these values correspond to the 5l WS 2 and MoS 2 bandgaps. We then examined the time-resolved photocurrent measurement using white-light illumination, as shown in Fig. 7e (result using specific laser wavelength is shown in Supplementary Fig. 14 ). The white light was first turned off for a period of 5 s, and then turned on for 5 s with the biasing V ds =5 V. The drain current ( I ds ) increased on activation of the light and decayed following removal of the incident light. The induced photocurrents were 39 pA, 13 pA and 11 pA for the VCC Mo 1− x W x S 2 multilayer, 5l WS 2 and 5l MoS 2 devices, respectively. Hence, the VCC Mo 1− x W x S 2 multilayer generates three to four times greater photocurrent than 5l WS 2 or 5l MoS 2 , which is attributed to broadband light absorption. Thus, we concluded that the VCC Mo 1− x W x S 2 multilayer is promising as regards use as an efficient photodetector with broadband light absorption. Furthermore, the broadband light absorption property is feasible for various optoelectronic applications such as solar cells [49] , [50] . In summary, we developed an ALD-based Mo 1− x W x S 2 synthesis process using sulfurization of super-cycle ALD Mo 1− x W x O y thin film. We studied the sulfurization process of ALD MoO x thin films to produce uniform and continuous MoS 2 . The synthesized ALD-based Mo 1− x W x S 2 alloy show good stoichiometry, uniform and continuous surfaces, controlled composition and layer numbers, and mixing of Mo and W atoms. Moreover, we developed a simple method to synthesize a VCC Mo 1− x W x S 2 multilayer with a clean interface, which shows stronger interlayer coupling than that of a stacked VCC Mo 1− x W x S 2 multilayer fabricated using the transfer process. Further, we have shown that the VCC Mo 1− x W x S 2 multilayer has promising potential applications as an efficient photodetector, because of its broadband light absorption capability. It should also be noted that the ALD-based TMDCs alloy synthesis process is not only limited to Mo 1− x W x S 2 , and we expect that similar process strategies can be developed for other TMDCs materials and their vertical stacks. MoO x film growth and characteristics A 6-inch ALD chamber containing a loadlock chamber was used for the deposition of the MoO x films. The films were deposited on SiO 2 (300 nm)/Si substrates by plasma-enhanced ALD using Mo(CO) 6 and O 2 plasma at a 200 °C growth temperature. The temperature of the bubbler containing Mo(CO) 6 was maintained at 35 °C to produce adequate vapour pressure, and vapourized Mo(CO) 6 molecules were transported into the chamber by pure argon (99.999%) carrier gas. The O 2 flow and plasma power were fixed at 300 s.c.c.m. and 200 W, respectively. An ALD cycle consists of four steps: Mo(CO) 6 precursor exposure ( t s ), Ar purging ( t p ), O 2 plasma reactant exposure ( t r ) and another Ar purging ( t p ). In the ALD MoO x process, the t s , t p and t r were fixed at 5 s, 12 s and 5 s, respectively. Optimization of the ALD MoO x process is described in the Supplementary Fig. 1 . Mo 1− x W x O y Film Growth MoO x and WO 3 ALD processes [27] were used to deposit Mo 1− x W x O y film using super-cycle ALD (as shown in Fig. 3a ) under the same chamber and deposition conditions described above for the ALD of MoO x . After 10 cycles of WO 3 ALD to address nucleation delay [27] , we conducted super-cycle ALD, which consists of n cycles of MoO x ALD and m cycles of WO 3 ALD. The detailed process steps are shown in Supplementary Table 1 . Sulfurization processes One-step process . To sulfurize the ALD MoO x , the sample was placed in the centre of a tube furnace (1.2 inch in diameter). Initially, the sample was heated at 200 °C for 60 min under flowing H 2 (25 s.c.c.m.) and Ar (25 s.c.c.m.) gas, to remove any organic contaminants on the surface. Subsequently, the temperature was gradually increased from 200 to 1,000 °C at 13.3 °C min −1 , and this temperature was then maintained for 60 min with flowing Ar (50 s.c.c.m.) and H 2 S (5 s.c.c.m.). Then, the sample was cooled to room temperature under a flowing Ar (50 s.c.c.m.) atmosphere. Two-step process . Initially, samples were annealed at 200 °C as in the one-step process. Then, the temperature was gradually increased from 200 °C to first-sulfurization temperatures of 600 or 800 °C at 13.3 °C min −1 . The peak temperature (600 or 800 °C) was maintained for 60 min with flowing Ar (50 s.c.c.m.) and H 2 S (5 s.c.c.m.). Subsequently, the temperature was gradually increased from the first-sulfurization temperatures to 1,000 °C at 13.3 °C min −1 and was maintained at this temperature for 30 min with flowing Ar (50 s.c.c.m.) and H 2 S (5 s.c.c.m.). The sample was cooled to room temperature under a flowing Ar (50 s.c.c.m.) atmosphere after the process was completed. Based on the results shown in Fig. 1 , we used a two-step sulfurization process with a 600 °C first-sulfurization temperature to sulfurize MoO x and Mo 1− x W x O y thin films in the MoS 2 and Mo 1− x W x S 2 alloy synthesis process. Transfer of MoS 2 and Mo 1− x W x S 2 The as-synthesized MoS 2 and Mo 1− x W x S 2 on the SiO 2 substrate were coated with polymethyl methacrylate (PMMA) by spin coating at 4,000 r.p.m. for 60 s. After curing of the PMMA at 100 °C for 15 min, the samples were immersed in 10% hydrogen fluoride solution to etch the SiO 2 layer. Subsequently, the samples were washed using deionized (DI) water and scooped onto a clean SiO 2 /Si substrate. The PMMA was removed by acetone and washed away using isopropyl alcohol. Characterization of MoS 2 and Mo 1− x W x S 2 OM (Olympus DX51), Raman spectroscopy (HORIBA, Lab Ram ARAMIS; 532-nm laser excitation wavelength), AFM (VEECO, Multimode), PL (SPEX1403, SPEX; 532-nm laser excitation wavelength), absorbance with ultraviolet–visible spectrophotometer (JASCO Corporation, V-650), XPS (Thermo UK, K-alpha), SEM (JEOL Ltd, JSM-6701F), TEM (FEI Titan G2 Cube 60-300; accelerating voltage, 80 kV), STEM and EDX (JEM 2100F; accelerating voltage, 200 kV) analyses were employed to characterize the MoS 2 and Mo 1− x W x S 2 alloy, and a VCC Mo 1− x W x S 2 multilayer. Fabrication and characterization of photodetectors Photodetectors were fabricated from an as-synthesized VCC Mo 1− x W x S 2 multilayer, 5l WS 2 and 5l MoS 2 on a SiO 2 (300 nm)/Si substrate by evaporating Au(40 nm)/Ti(1 nm) electrodes with 100-μm channel length. Electrical measurements were conducted using a Keithley 2400 (Keithley Instruments). The photocurrent was measured by modulating the laser beam with a mechanical chopper (1,000 Hz) and detecting the photocurrent with a current preamplifier and a lock-in amplifier. A monochromator was used for wavelength-dependent measurements of the photocurrent. Parameters for analysis of XPS and Raman We used Spectral Data Processor v4.1 for the XPS and Raman spectra fitting. In the fitting analysis of the XPS spectra, the full widths at half maximum (FWHM) were between 1.7 and 1.9 eV, the Lorentzian Gaussian Ratio was 2:8, the energy difference between the Mo3d spin-orbit doublet was set to 3.2 eV and the branching ratio was 2/3. In addition, we used Scofield Relative Sensitivity Factor for calculation of stoichiometry as represented in Supplementary Table 2 . For the Raman spectrum fitting analysis, the FWHM was between 7 and 12 cm −1 . How to cite this article: Song, J. G. et al . Controllable synthesis of molybdenum tungsten disulfide alloy for vertically composition-controlled multilayer. Nat. Commun. 6:7817 doi: 10.1038/ncomms8817 (2015).